Whole-genome sequencing ofOryza brachyanthareveals mechanisms underlyingOryzagenome evolution The wild species of the genus Oryza contain a largely untapped reservoir of agronomically important genes for rice improvement. Here we report the 261-Mb de novo assembled genome sequence of Oryza brachyantha . Low activity of long-terminal repeat retrotransposons and massive internal deletions of ancient long-terminal repeat elements lead to the compact genome of Oryza brachyantha . We model 32,038 protein-coding genes in the Oryza brachyantha genome, of which only 70% are located in collinear positions in comparison with the rice genome. Analysing breakpoints of non-collinear genes suggests that double-strand break repair through non-homologous end joining has an important role in gene movement and erosion of collinearity in the Oryza genomes. Transition of euchromatin to heterochromatin in the rice genome is accompanied by segmental and tandem duplications, further expanded by transposable element insertions. The high-quality reference genome sequence of Oryza brachyantha provides an important resource for functional and evolutionary studies in the genus Oryza . Comparative genomics based on the fully sequenced genomes of model organisms have gained insights into gene and genome evolution [1] , [2] , [3] . In plants, the genome organization was perplexed by whole-genome duplication, transposable elements and sequence rearrangements [1] , [4] . Even closely related species, such as species in the genus Arabidopsis or Oryza , harbour remarkable fluctuations in genome size, gene number and gene collinearity [5] , [6] . So far, the completely sequenced plant genomes are mostly within a long-range evolutionary timeframe [2] , thus limiting the ability to deduce the underlying mechanisms for genomic changes. Instead, comparative analysis of orthologous regions or whole-genome sequences within a short evolutionary timeframe, especially within the same genus, brings novel insights into the nature, rate and mechanisms of genome rearrangements [5] , [6] , [7] , [8] , [9] . The genus Oryza , consisting of 24 species along an evolutionary gradient of ~15 million years, is an ideal model for studying plant genome evolution [10] , [11] , [12] . The evolutionary signatures of Oryza genome evolution vary among different loci [6] , [13] , [14] , suggesting the demand for whole-genome comparisons of these Oryza species. The wild rice Oryza brachyantha is defined as F genome type and placed on the basal lineage in Oryza [15] ( Supplementary Note S1 and Supplementary Fig. S1 ). It contains a different set of repeat sequences compared with rice or other Oryza genomes [16] , [17] . Its compact genome and unique phylogenetic position put O. brachyantha more close to the ancestral state of the Oryza genomes [10] ( Supplementary Note S1 and Supplementary Figs S1 and S2 ). Thus, comparisons of the O. brachyantha and rice genomes will provide us a unique opportunity to explore the genomic changes and the underlying mechanisms of Oryza genome evolution. We used a whole-genome shotgun approach combined with the bacterial artificial chromosome (BAC)-based physical map to assemble ~261 Mb of the O. brachyantha genome. O. brachyantha has a compact genome composed of less than 30% of repeat elements. We annotated 32,038 gene models in O. brachyantha , which is much lower than in rice [18] , implying a massive amplification of gene families in the domesticated rice genome. We showed that both tandem gene duplications and gene transpositions had contributed to the burst of gene families in the rice genome. These duplicated sequences might have impacts on the erosion of synteny and accumulation of transposable elements in the heterochromatic regions. Sequence and assembly We used a whole-genome shotgun sequencing approach to generate 31 Gb of the raw sequence of O. brachyantha using the Illumina GA II platform ( Supplementary Table S1 ). The genome was initially assembled using SOAP denovo [19] , and the length of the sequence scaffold was further increased by integrating BAC-end sequences generated by Sanger technology [20] ( Supplementary Methods ). The final assembled sequence was 261 Mb with a scaffold N50 size of 1.6 Mb ( Supplementary Table S2 ). The ordering of the scaffolds along each chromosome was accomplished by integration with the BAC-based physical map [20] . The scaffolds were eventually merged into 36 large sequence blocks covering 96% of the sequenced genome ( Fig. 1 ). These sequence blocks were anchored onto each chromosome by a cytogenetic approach ( Supplementary Fig. S3 ), resulting in 12 pseudomolecules representing the 12 chromosomes of O. brachyantha . 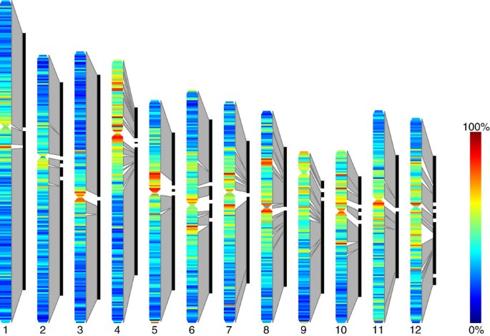Figure 1: Alignment of 36 sequence blocks ofO. brachyanthato rice chromosomes. Rice chromosomes are shown on the left, filled with density of repeat elements for every 100 kb window. Sequence blocks ofO. brachyanthaon each chromosome are represented by black boxes on the right. Syntenic regions, defined as described in Methods, are shaded in grey. Large sequence blocks were anchored to the chromosomes by a cytogenetic approach. Small sequence blocks of pericentromeric regions, in which few collinear genes could be defined, were anchored to the chromosomes by integration with the physical map and confirmation by Southern blot. Figure 1: Alignment of 36 sequence blocks of O. brachyantha to rice chromosomes. Rice chromosomes are shown on the left, filled with density of repeat elements for every 100 kb window. Sequence blocks of O. brachyantha on each chromosome are represented by black boxes on the right. Syntenic regions, defined as described in Methods, are shaded in grey. Large sequence blocks were anchored to the chromosomes by a cytogenetic approach. Small sequence blocks of pericentromeric regions, in which few collinear genes could be defined, were anchored to the chromosomes by integration with the physical map and confirmation by Southern blot. Full size image Transposable elements in O. brachyantha Approximately 29.2% of the O. brachyantha genome is composed of transposable elements ( Supplementary Table S3 ), lower than rice [18] (34.8%), sorghum [21] (62.0%) and maize [22] (84.2%), consistent with their genome sizes. The Mutator -like element is the most abundant transposon family, accounting for 7.5% (18.3 Mb versus 13.4 Mb in rice [18] ) of the O. brachyantha genome and more than 25% of the DNA transposons in O. brachyantha . Retrotransposons, mostly long-terminal repeat (LTR) retrotransposons, comprise ~10% of the O. brachyantha genome. A total of 184 LTR retrotransposon families have been discovered, including 75 Ty1- copia , 55 Ty3- gypsy and 54 unclassified families. It is interesting to note that 40 families are present in the form of solo LTRs or fragments. The transposable elements are unevenly distributed on each chromosome with retrotransposons concentrated in pericentromeric or heterochromatic regions ( Fig. 2 and Supplementary Fig. S4 ). 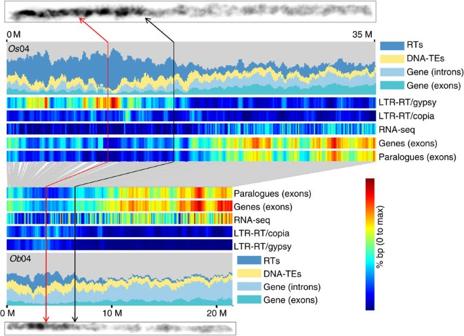Figure 2: Distributions of genomic features inO. brachyanthaandO. sativaon chromosome 4. The twoOryzagenomes showed similar distributions of gene and repeat elements: DNA transposons (DNA-TEs) showed a relatively even distribution along the chromosomes, whereas retrotransposons (RTs) were negatively correlated with the distribution of genes. The overall level of RTs was higher inO. sativathan inO. brachyantha, in which the short arms and the proximal regions of the long arms of chromosome 4 showed much obvious contrast. These highly repetitive regions also showed reduced levels of transcription and gene collinearity. The 4',6-diamidino-2-phenylindole-stained pachytene chromosomes forO. brachyanthaandO. sativawere put along the genomic tracks of chromosome 4. The black arrows indicate the transition region of euchromatin/heterochromatin, whereas the red arrows indicate the centromere positions. Figure 2: Distributions of genomic features in O. brachyantha and O. sativa on chromosome 4. The two Oryza genomes showed similar distributions of gene and repeat elements: DNA transposons (DNA-TEs) showed a relatively even distribution along the chromosomes, whereas retrotransposons (RTs) were negatively correlated with the distribution of genes. The overall level of RTs was higher in O. sativa than in O. brachyantha , in which the short arms and the proximal regions of the long arms of chromosome 4 showed much obvious contrast. These highly repetitive regions also showed reduced levels of transcription and gene collinearity. The 4',6-diamidino-2-phenylindole-stained pachytene chromosomes for O. brachyantha and O. sativa were put along the genomic tracks of chromosome 4. The black arrows indicate the transition region of euchromatin/heterochromatin, whereas the red arrows indicate the centromere positions. Full size image The evolution of genome size in Oryza The genomic comparison revealed that only 35% of the O. brachyantha genome was conserved with the rice genome ( Supplementary Fig. S5 ). The genome size variation between the O. brachyantha and rice genomes was mainly caused by differences in the lineage-specific evolution of intergenic sequences, of which LTR retrotransposons alone contributed to ~50% of the size difference ( Supplementary Figs S5 and S6 ). In O. brachyantha , the amplification of LTR retrotransposons occurred over a relatively long period, with a peak of activity approximately two to three million years ago (MYA; Fig. 3a ). Only 5.2% of the LTR retrotransposons were amplified more recently (that is, over a period of less than 0.5 MYA). In contrast, nearly 40% of the LTR retrotransposons were inserted into the rice genome within the last 0.5 million years. Consistent with earlier findings [23] , two recent bursts were observed in the rice genome (<0.5 and 1–2 MYA), which together represent 70% of the LTR retrotransposons in rice ( Fig. 3a ). These results indicate that massive recent amplifications of LTR retrotransposons, as occurred in maize [22] and sorghum [21] , expanded the rice genome in the last two million years. 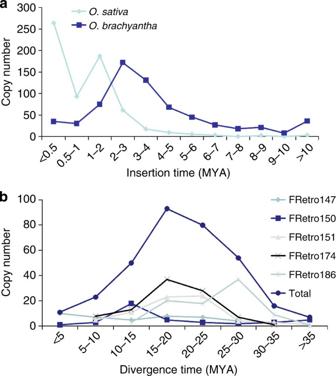Figure 3: Dynamic evolution of LTR retrotransposon inO. brachyanthaandO. sativa. (a) Insertion time of LTR retrotransposons in theO. brachyanthaand rice genomes. For comparison, LTR retrotransposons of rice chromosomes 3 and 8 were annotated using the same method described forO. brachyantha. The insertion times of LTR retrotransposons were estimated from intact LTR retrotransposons as described in Methods. (b) Divergence time of solo LTR families inO. brachyantha. The divergence times of five families with only solo LTR members were estimated as described in Methods. Figure 3: Dynamic evolution of LTR retrotransposon in O. brachyantha and O. sativa . ( a ) Insertion time of LTR retrotransposons in the O. brachyantha and rice genomes. For comparison, LTR retrotransposons of rice chromosomes 3 and 8 were annotated using the same method described for O. brachyantha . The insertion times of LTR retrotransposons were estimated from intact LTR retrotransposons as described in Methods. ( b ) Divergence time of solo LTR families in O. brachyantha . The divergence times of five families with only solo LTR members were estimated as described in Methods. Full size image To counteract the expansion, LTR retrotransposons could be eliminated from the genome through unequal homologous recombination or non-homologous (illegitimate) recombination, resulting in solo LTRs or truncated LTR retrotransposons [24] , [25] . The results of higher ratios of solo LTRs and truncated elements to intact LTR elements in O. brachyantha than rice suggests a tendency of shrinkage in O. brachyantha (solo: intact LTR of 1.63 in O. brachyantha versus 0.93 in rice, and truncated: intact LTR of 3.26 in O. brachyantha versus 0.64 in rice). The divergence times of the five solo LTR families indicate that these elements are likely to be ancient families in the genus Oryza , being inactive by deletions, and eventually will be removed from the genome of O. brachyantha by sequence decay ( Fig. 3b and Supplementary Table S4 ). These results are consistent with recent findings in Arabidopsis that deletion was selectively favoured in a compact genome, in which repression of transposable elements is more efficient [5] , [26] . Thus, we conclude that limited recent activity and a massive removal of ancient families through unequal homologous recombination and illegitimate recombination have led to the smaller genome size of O. brachyantha . Evolution of gene families in Oryza A total of 32,038 protein-coding genes were predicted in O. brachyantha using an evidence-based strategy [27] ( Supplementary Methods ). In 18,020 gene families of O. brachyantha , 17,076 (95%) are clustered with rice genes ( Fig. 4 ). More than 80% of the gene families shared by O. brachyantha and rice have a one-to-one orthologous relationship. Moreover, 1,419 families have a smaller size in O. brachyantha , whereas only 460 families are of a smaller size in rice ( Fig. 5a ). Analysis of the Pfam domains indicates that the gene families, such as NB-ARC ( P -value ≤1.05 × 10 −5 ), Leucine-rich repeat (LRR, P -value≤2.20 × 10 −16 ) and F-box ( P -value ≤2.20 × 10 −16 ), are overrepresented in rice relative to O. brachyantha ( Fig. 5b and Supplementary Methods ). These disease resistance-related gene families are evolved at a high birth- and death rate in plant genomes, which may reflect its role in adaptation to various environments [5] , [28] . Further exploration of gene families of NBS–LRR and RLK–LRR suggests remarkable turnover of family members through gene duplication, transposition and pseudogenization [29] ( Supplementary Methods , Supplementary Tables S5–S8 and Supplementary Figs S7–S10 ). 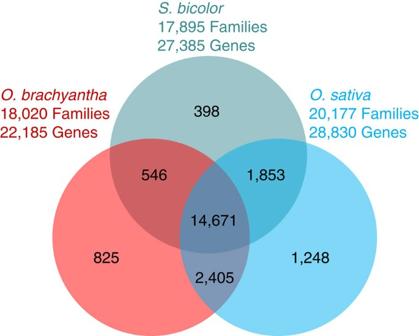Figure 4: Venn diagram showing the distribution of gene families betweenO. brachyantha,O. sativaandSorghum bicolor. Orthologous gene families are defined in Methods. The numbers of gene families and genes clustered in families are indicated for every species. The intersections between species indicate the numbers of shared gene families, whereas the numbers of unique families are shown in species-specific areas. Figure 4: Venn diagram showing the distribution of gene families between O. brachyantha , O. sativa and Sorghum bicolor . Orthologous gene families are defined in Methods. The numbers of gene families and genes clustered in families are indicated for every species. The intersections between species indicate the numbers of shared gene families, whereas the numbers of unique families are shown in species-specific areas. 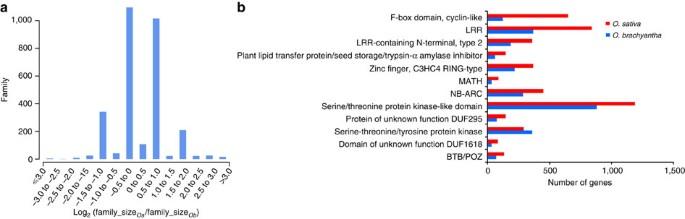Figure 5: Comparison of gene families betweenO. brachyanthaandO. sativa. (a) Size variation of gene families. All shared gene families betweenO. brachyanthaandO. sativa, excluding one-to-one orthologues, were compared to show the variation in gene family sizes. Negative values indicate fewer family members inO. sativa, whereas positive values indicate more members inO. sativa.Os,O. sativa;Ob,O. brachyantha. (b) Copy number variation of conserved functional domains. The gene number belonging to each conserved functional domain was retrieved according to Pfam domain annotation (Methods). Theχ2-test, or Fisher’s exact test when the expected frequency was smaller than five, was employed to select significantly different functional domains betweenO. brachyanthaandO. sativa. Multiple comparisons were corrected by the Bonferroni method as implemented in R. Only significant functional domains with a total number of more than 100 members in twoOryzagenomes are shown, ranked byP-value (P-value ≤2 × 10−4andq-value ≤0.05). Full size image Figure 5: Comparison of gene families between O. brachyantha and O. sativa . ( a ) Size variation of gene families. All shared gene families between O. brachyantha and O. sativa , excluding one-to-one orthologues, were compared to show the variation in gene family sizes. Negative values indicate fewer family members in O. sativa , whereas positive values indicate more members in O. sativa . Os , O. sativa ; Ob , O. brachyantha . ( b ) Copy number variation of conserved functional domains. The gene number belonging to each conserved functional domain was retrieved according to Pfam domain annotation (Methods). The χ 2 -test, or Fisher’s exact test when the expected frequency was smaller than five, was employed to select significantly different functional domains between O. brachyantha and O. sativa . Multiple comparisons were corrected by the Bonferroni method as implemented in R. Only significant functional domains with a total number of more than 100 members in two Oryza genomes are shown, ranked by P -value ( P -value ≤2 × 10 −4 and q -value ≤0.05). Full size image Conservation of gene organization along chromosomes in Oryza The gene organization of Oryza species is highly conserved as demonstrated by regional sequence analysis, although exceptions have been observed [6] , [13] , [14] . To reveal the degree and nature for genome organization changes between rice and O. brachyantha separated in evolution for approximately 15 million years, we performed a whole-genome collinearity analysis. Core-orthologous gene pairs were used to define 82 orthologous blocks between the O. brachyantha and rice genomes, which covered ~97% ( O. brachyantha ) and 94% (rice) of predicted gene models. The break intervals between orthologous blocks, including 11 centromeres, were formed by long stretches of nonsyntenic genomic sequences in one or both genomes ( Fig. 1 ). On the basis of the syntenic blocks, we found 22,405 and 24,103 genes that were conserved in gene collinearity between O. brachyantha and rice, respectively. These collinear gene pairs formed 19,222 gene clusters, 2,468 of which showed evidence of local gene duplications ( Fig. 6 ). We found many more expanded clusters in rice than that in O. brachyantha (1,363 and 663, respectively). Analysis of functional categories revealed that the duplicated genes were enriched in defence and reproduction process categories, which was consistent with the gene family analysis and suggested significant roles of local duplications in these gene families ( Supplementary Table S9 ). We identified 214 inversions between O. brachyantha and rice genomes ( Fig. 6 and Supplementary Figs S11 and S12 ). Approximately two-thirds of the inversions were flanked by inverted repeat sequences in one or both genomes; two inversions in the rice genome were found to be linked with the duplication of a flanking gene, revealing a potential novel mechanism for gene duplication [30] , [31] ( Supplementary Figs S13 and S14 , and Supplementary Table S10 ). 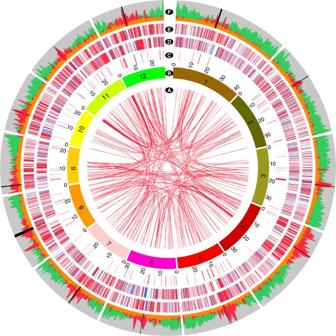Figure 6: Distribution of sequence rearrangements along the chromosomes ofO. sativa. Segmental duplications, tandem duplications, inversions and non-collinear sequence blocks were detected as described in Methods. (a), Donors and acceptors of segmental duplications on rice chromosomes are connected by red lines. (b), Chromosome ideograms in the inner circle are represented by different colours, with chromosome numbers indicated. The three internal heatmaps represent inversions (c), expansion of tandem gene duplications (d) and expansion of non-collinear sequence blocks (e), in which expansion in rice is indicated by red colour and expansion inO. brachyanthaindicated by blue colour. Of the 214 inversions betweenO. brachyanthaand rice genomes, only inversions with more than two collinear genes are shown. Of the 2,460 orthologous tandem gene clusters, 1,378 tandem clusters expanded in the rice genome are shown as red colour and 654 tandem clusters expanded inO. brachyanthaare shown as blue colour. Of the non-collinear sequence blocks, only those regions that had expanded more than double in size in rice orO. brachyanthaare shown in red or blue, respectively. (f), The densities of genes, RNA retrotransposons and DNA transposons are shown as green, red and orange histograms in the outer circle, respectively. Min–Max: gene (0–25%); RNA retrotransposon (0–80%); DNA transposon (0–80%). Centromeres are indicated by black bars in the outer circle. Figure 6: Distribution of sequence rearrangements along the chromosomes of O. sativa . Segmental duplications, tandem duplications, inversions and non-collinear sequence blocks were detected as described in Methods. ( a ), Donors and acceptors of segmental duplications on rice chromosomes are connected by red lines. ( b ), Chromosome ideograms in the inner circle are represented by different colours, with chromosome numbers indicated. The three internal heatmaps represent inversions ( c ), expansion of tandem gene duplications ( d ) and expansion of non-collinear sequence blocks ( e ), in which expansion in rice is indicated by red colour and expansion in O. brachyantha indicated by blue colour. Of the 214 inversions between O. brachyantha and rice genomes, only inversions with more than two collinear genes are shown. Of the 2,460 orthologous tandem gene clusters, 1,378 tandem clusters expanded in the rice genome are shown as red colour and 654 tandem clusters expanded in O. brachyantha are shown as blue colour. Of the non-collinear sequence blocks, only those regions that had expanded more than double in size in rice or O. brachyantha are shown in red or blue, respectively. ( f ), The densities of genes, RNA retrotransposons and DNA transposons are shown as green, red and orange histograms in the outer circle, respectively. Min–Max: gene (0–25%); RNA retrotransposon (0–80%); DNA transposon (0–80%). Centromeres are indicated by black bars in the outer circle. Full size image Mechanisms on erosion of gene collinearity The degree of gene collinearity in plant genomes tends to decrease with the increase of phylogenetic distance [4] , [32] , leaving less than 15% of rice genes collinear with eudicots and ~57% of rice genes collinear with sorghum. However, the underlying mechanism for non-collinear gene formation was not well understood [8] , [33] . We observed more than 30% of genes in O. brachyantha or rice are located in non-collinear positions, with more than half of them supported by homologous proteins or transcriptome data ( Supplementary Table S11 ). These non-collinear genes were enriched in pericentromeric or heterochromatic knobs than euchromatic regions in the rice genome, resulting reduced level of gene collinearity in these recombination-inert regions ( Supplementary Figs S15 and S16 ). To reveal the mechanism by which non-collinear genes were created, we introduced an intermediate species Oryza glaberrima , which diverged from rice less than 2 MYA [12] . We identified 198 non-collinear genes accumulated in the rice genome posterior to its split with O. glaberrima , including 127 insertions. Forty-five per cent (56 insertions) of them were found to have highly identical homologues in the rice genome ( Supplementary Table S12 ). By comparison of these 56 trisequence alignments among non-collinear gene regions (acceptor sites), their closest homologous regions (donor sites) and their orthologous regions in Oryza glaberrima (putative ancestral sites), the mechanisms by which the non-collinear genes were created can be revealed ( Fig. 7 and Supplementary Figs S17 and S18 ). Transposable elements, which have been shown to be frequently involved in gene movements in plant genomes [34] , were found to dominate in 12 insertions ( Supplementary Table S12 ). In three cases, we observed that the acceptor sites have long stretches of homologous sequences with the donor sequence, suggesting the insertions were caused by non-allelic homologous recombination during repair of double-strand breaks [35] ( Fig. 7b (III) and Supplementary Fig. S17c ). However, in 41 cases the comparisons revealed no signature of transposable elements or long homologous sequence, but showed microhomology (<10 bp) between the flanking sequences of the acceptor sites and the donor sites ( Supplementary Table S12 ). The sequence signatures suggest the insertions were associated with the repair of double-strand breaks through non-homologous recombination, including non-homologous end joining (NHEJ) and microhomology-mediated end joining [36] . The breakpoints of these 41 insertions in the rice genome were mostly precise without deletions when compared with O. glaberrima , thus indicating the role of NHEJ in creating these non-collinear genes [36] . The mechanisms of repair of double-strand breaks through non-homologous recombination or non-allelic homologous recombination had important roles in structure variations of human genomes [37] , [38] . Our findings suggest that the repair of double-strand breaks, particularly NHEJ, has a dominant role in gene duplications, and in creating synteny perturbations in plant genomes. 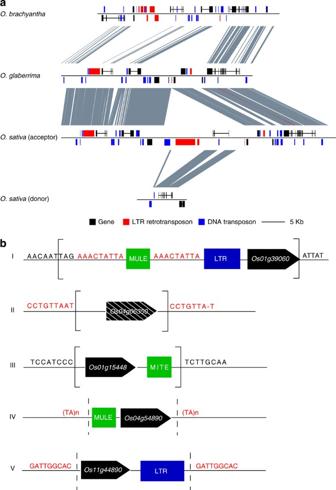Figure 7: Genomic rearrangements and signature of breakpoints. (a) Sequence analysis of a non-collinear gene locus. The region containing an expansion on chromosome 1 ofO. sativawas compared with orthologous regions inO. brachyanthaandO. glaberrima. Nearly 17.2 kb of the expansion inO. sativa(acceptor) was formed by an insertion after its split withO. glaberrima. The insertion sequence was highly homologous to a genomic segment on chromosome 9 ofO. sativa(donor). Analysis of the breakpoints indicated that the acceptor sequence was a duplicated copy of the donor sequence. (b) Molecular signatures of recently formed non-collinear genes. Red characters, target site duplication; black arrowhead boxes, genes; shaded black arrowhead boxes, pseudogenes; blue boxes, LTR retrotransposons; green boxes, DNA transposons; orange boxes, non-LTR retrotransposons; sequences between square brackets have highly homologous donor sequences; sequences between dashes have no donor sequences. Detailed sequence analyses are shown inSupplementary Figs S17 and S18. MULE,Mutator-like element. Figure 7: Genomic rearrangements and signature of breakpoints. ( a ) Sequence analysis of a non-collinear gene locus. The region containing an expansion on chromosome 1 of O. sativa was compared with orthologous regions in O. brachyantha and O. glaberrima . Nearly 17.2 kb of the expansion in O. sativa (acceptor) was formed by an insertion after its split with O. glaberrima . The insertion sequence was highly homologous to a genomic segment on chromosome 9 of O. sativa (donor). Analysis of the breakpoints indicated that the acceptor sequence was a duplicated copy of the donor sequence. ( b ) Molecular signatures of recently formed non-collinear genes. Red characters, target site duplication; black arrowhead boxes, genes; shaded black arrowhead boxes, pseudogenes; blue boxes, LTR retrotransposons; green boxes, DNA transposons; orange boxes, non-LTR retrotransposons; sequences between square brackets have highly homologous donor sequences; sequences between dashes have no donor sequences. Detailed sequence analyses are shown in Supplementary Figs S17 and S18 . MULE, Mutator -like element. Full size image Impact of duplications on the evolution of chromatin Duplicated sequences were found frequently in, but were not restricted to, heterochromatic regions, consistent with their important role in accumulating non-collinear genes in these regions [39] ( Fig. 6 ). Owing to their redundancy, these duplications were more tolerant of mutations, such as transposon insertions and sequence rearrangements, and may therefore act as a hotspot for genome expansion [40] . If this is the case, we would expect much more expansions in these duplication-rich regions. Indeed, sequence rearrangements were distributed across all of the chromosomes with a particular concentration in the pericentromeric and heterochromatic regions ( Fig. 6 and Supplementary Fig. S19 ). In contrast to the collinear regions, the rearranged regions displayed more differences in size between O. brachyantha and rice, with more regions expanded in rice than in O. brachyantha ( Fig. 6 and Supplementary Fig. S19 ). More specifically, we observed a much greater expansion in rice heterochromatic regions H7 and H8 on chromosome 4 ( Table 1 and Supplementary Figs S20 and S21 ), even with a lower abundance of LTR retrotransposons (29 and 24%). In both regions, gene duplication had a substantial role in genome expansion. Seven tandemly duplicated gene clusters were found in the H8 region, which contributed to ~726 kb expansion in rice ( Supplementary Fig. S21 ). Besides tandem duplications, segmental duplications comprised 137 kb of extra sequences in the H7 region of rice ( Supplementary Fig.S20 ). We also found the rate of retrotransposon accumulation was increased in the duplicated regions of H1 heterochromatic region on chromosome 4, resulting in a very high level of expansion in rice ( Table 1 and Supplementary Fig. S22 ). These results were consistent with the cytogenetic observations that the proximal region of the long arm of rice chromosome 4 were highly heterochromatic, but condense of chromatin were almost undetectable in O. brachyantha ( Fig. 2 ). The evolutionary fluidity of euchromatin and heterochromatin in orthologous regions between closely related species were also observed in Drosophila , which showed potential influence on gene regulation, implying important roles in species divergence [41] , [42] . The phenomena for transposable element accumulations in duplicated sequences suggest an important role of duplication in genome expansion, and possibly in the formation of heterochromatin [40] . Table 1 Comparative analysis of orthologous sequences in heterochromatic domains between O. brachyantha and O. sativa. Full size table Understanding the gene and genome evolution needs both within- and between-species comparisons. The studies in Drosophila , yeast and human lineages demonstrated how comparisons on genome sequences of closely related species revealed mechanisms on gene and genome evolution in animals [7] , [9] , [43] . In plants, Oryza is an excellent system for comparative genomics [6] , [13] . The genomic recourses of Oryza were well developed, including BAC libraries and fingerprinted physical maps [20] . An international Oryza Map Alignment Project is on the way to generate reference genome sequences for ten representative species in Oryza [44] . O. brachyantha is of importance because it is one of the most diverged wild rice species and the genome is likely to be more static compared with other Oryza genomes; thus, this provides an opportunity to explore the signatures of gene and genome evolution of Oryza by comparing with the rice genome. Taking advantage of the BAC-based physical map, we produced a high-quality genome sequence of O. brachyantha , of which 96% was assembled into 12 pseudo-chromosomes. By manual annotation of the repeat sequences, we demonstrated that the genome of O. brachyantha is more stable with limited activity of transposable element amplifications. The gene number is comparable to that of sorghum [21] , Brachypodium [45] and rice [18] . However, through detailed analysis on gene collinearity we found that the rice genome experienced a massive gene amplification after the divergence of Oryza . Besides the contribution of tandem gene duplications, most gene amplifications were caused by gene transpositions that copy and paste genes to non-collinear positions. The gene transposition could be very critical to evolution if the resulting gene evolved towards a novel function or caused interspecies incompatibility. For example, one gene transposition (LOC_OS01g15448, DPL1 ), caused by non-allelic homologous recombination through double-strand break repair, together with its parental gene (LOC_OS06g08510, DPL2 ), are responsible for the hybrid incompatibility between indica and japonica rice through reciprocal gene loss [46] . Several mechanisms were proposed to underlie the formation of non-collinear genes, including capture of gene fragments by transposable elements, retroposition and double-strand break repair [33] . The analysis of this study suggested that NHEJ through double-strand break repair accounts for most cases of gene transpositions in the rice genome. The breakpoints of gene transpositions were precisely determined by comparing the flanking sequences with the donor sites. The repair process needs very few homologous sequences or can occur without homologous sequences, implying even distribution along the chromosomes. However, non-collinear genes were found to be significantly enriched in heterochromatic regions, suggesting that the repression of recombination in heterochromatin might not be efficient in removing non-collinear genes in these regions. The accumulation of duplicated sequences resulted in the complexity of genome organization in heterochromatin. In addition, these redundant sequences are tolerant of transposable element insertions, thus facilitate the accumulation of transposable elements resulting in the transition from euchromatin to heterochromatin. A recent study reported a de novo assembly of the wild ancestor of cultivated rice, O. rufipogon [47] . Comparing the genome sequence with the rice genome revealed many functional structure variants located in domestication loci in rice, suggesting possible roles of functional variants in rice domestication [47] . In summary, we generated a high-quality de novo reference genome sequence of O. brachyantha . Comparisons with the rice genome revealed mechanisms underlying genome size variation, gene family expansion, gene movement and transition of euchromatin to heterochromatin in the Oryza genomes. Future whole-genome sequencing of the collective Oryza genomes along an evolutionary gradient will render the genus Oryza an unparalleled system for functional and evolutionary studies in plants. Sequence and assembly The plants of O. brachyantha (IRGC101232) were kindly provided by the International Rice Research Institute. The nuclear DNA of O. brachyantha was isolated from young leaves using a modified cetyl trimethylammonium bromide protocol, followed by purification using phenol–chloroform. The genomic DNA was fragmented into different sizes to prepare pair-end libraries using standard Illumina protocols. Sequencing was performed on an Illumina Genome Analyzer II. The BAC library and physical map of O. brachyantha was constructed by the Oryza Map Alignment Project at the Arizona Genomics Institute. The sequence assembly was performed with SOAP denovo [19] . Reconstruction of pseudo-chromosomes was accomplished by integrating the scaffold sequences with the physical map and confirmed by cytogenetic approaches. Complete details are described in Supplementary Methods . Gene annotation Protein-coding genes were predicted with the Gramene Genebuilder using a strategy of evidence-based gene prediction [27] ( Supplementary Methods ). FGENESH was used to improve the evidence-based gene models and add further models that had been missed by Gramene Genebuilder. Protein and transcriptional data were collected from various plant species, with a particular focus on monocot species ( Supplementary Methods ). The translated coding sequences were obtained from four sequenced monocot species, as well as Poplar and Arabidopsis ( Supplementary Methods ). The full-length complementary DNAs were obtained mainly from rice (50%) and maize (36%). We also included RNA-seq transcripts from O. brachyantha to improve the accuracy of the gene prediction. Protein-coding genes were annotated by InterProScan to assign Pfam domains and Gene Ontology annotations [48] . Orthologous gene families among O. brachyantha , O. sativa (TIGR6.1) and S. bicolor (v1.4) were identified by OrthoMCL [49] based on BLASTP results with E -values of 10 −5 . The genome assembly, annotation and genome browser can be found at http://www.gramene.org/Oryza_brachyantha . Repeat annotation A custom repeat library was developed for O. brachyantha based on structure signatures of different repeat families, as well as homologous searches to known repeat libraries ( Supplementary Methods ). LTR retrotransposons were detected by screening the genome of O. brachyantha with LTR-Finder [50] . Solo LTRs were discovered by combining analysis of homologous sequence, target site duplication and terminal motif of LTR. Non-LTR retrotransposons and DNA transposons were detected by searching the genome with conserved domains of each repeat family. The candidate sequences were manually checked for the structure signals and target site duplication as described in the Supplementary Methods . Classification of subfamilies was based on 80–80–80 rules for LTR retrotransposons and Mutator -like element transposons [51] . Estimation of the insertion times for LTR retrotransposons To estimate the insertion times for the full-length LTR retrotransposons, the 5′- and 3′-LTR sequences of the retrotransposons were aligned and used to calculate the K -value (the average number of substitutions per aligned site) using the MEGA 4 programme [52] . The insertion times ( T ) were calculated using the formula: T = K /(2 × r ), where r represents the average substitution rate, which is 1.3 × 10 −8 substitutions per synonymous site per year [53] . To estimate the divergence date of the retrotransposons that are present in the genome as solo LTRs only, all the intact solo LTRs in the family were used to build a phylogenetic tree and to generate a consensus based on the sequence alignments between the copies of a cluster. All copies of the family were then aligned with the consensus to calculate the K -value. The divergence time was estimated using the same formula and r -value as described above. Tandem duplication and segmental duplication Tandem duplication was defined as neighbouring genes that were not interrupted by more than ten genes. Protein-coding genes were self-searched with E -values ≤10 −5 . The homologous genes were used to construct an undirected graph. Gene pairs in the graph that had a distance of more than ten genes were filtered out. Tandem gene clusters were then retrieved based on resulting connections in the graph. LASTZ was used to identify segmental duplications (length ≥5 kb; identity ≥90%) in O. sativa [54] . All self-match alignments were detected by LASTZ based on the repeat-masked genome of O. sativa ( K =2,200, L =6,000, Y =3,400, E =30, H =0, O =400, T =1). The original alignments were processed using the Chain/Net package [55] to chain the well-defined neighbouring alignments. The masked repeat sequences were then reintroduced to the alignments to obtain an optimal global alignment. The candidate segmental duplications (length ≥5 kb; identity ≥90%) were filtered to contain less than 70% repetitive sequences. Genes included in the segmental duplication were obtained by comparing the position of the segmental duplication with the annotated gene. Interspecies whole-genome alignment The genome sequence of O. brachyantha was masked by RepeatMasker using a custom repeat library created in this study. The genome sequence of O. sativa was masked by RepeatMasker using a rice repeat library. Tandem repeats were masked in both genomes using Tandem Repeat Finder [56] . The whole-genome alignment between O. brachyantha and O. sativa was constructed on masked genomes using LASTZ [54] with parameters: K =2,200, L =6,000, Y =3,400, E =30, H =0, O =400, T =1. Post-processing was performed using the Chain/Net package [55] with custom Perl scripts, resulting in a set of orthologous alignments. Gene collinearity and sequence rearrangements The syntenic blocks between O. brachyantha and O. sativa were defined by MCscan [4] based on core-orthologous gene sets identified using InParanoid [57] (BLAST E -value ≤10 −5 ; number of genes required to call synteny ≥5). The syntenic blocks were confirmed to represent the orthologous blocks between O. brachyantha and O. sativa. Genes were then classified as collinear or non-collinear according to whether they have a homologous gene in the orthologous regions. If a homologous gene was not detected in the syntenic region of the target genome, we would search for homologous DNA sequences of the candidate gene in this region and syntenic status would be assigned ‘without synteny status’ for this gene when sequence remnants was detected, which means the orthologous gene was probably missannotated and the synteny status of this gene is not sure. To minimize the influence of sequence gaps on synteny analysis, we manually inspected the gap-containing genes and gap-flanking genes to confirm their syntney status and incorporate the result into synteny analysis. We also used sorghum [21] , Brachypodium [45] and foxtail millet [58] as outgroups to filter these candidate non-collinear genes that were collinear with outgroups. The same procedure was performed between O. sativa and O. glaberrima genomes, which was provided by Dr Rod Wing, to get the most recently formed non-collinear genes in the rice genome. A collinear region is described as a region that contains only collinear genes in both genomes, whereas a rearranged region is described as a region that contains only non-collinear genes or sequence arrangements, such as inversions, in both genomes. Inversions are defined as a region or a cluster of genes that is shared between O. brachyantha and rice, but in the reverse direction. The 10-kb sequences flanking inversions were compared by SSEARCH [59] to find inverted repeats between the upstream and downstream sequences of inversions ( E -value ≤0.01), which could cause inversions by homologous recombination. Gene expressions of duplicated genes were obtained from the Rice MPSS database [60] . Accession codes: The raw reads for this project have been deposited in the NCBI SRA project under the accession number SRA046388 . The Illumina reads can be accessed under SRX099337 to SRX099351 for whole-genome shotgun reads and SRX100097 to SRX100098 for RNA-seq reads. The genome assembly has been deposited in DDBJ/EMBL/GenBank under the accession AGAT00000000 . The version described in this paper is the first version, AGAT01000000 . How to cite this article: Chen, J. et al . Whole-genome sequencing of Oryza brachyantha reveals mechanisms underlying Oryza genome evolution. Nat. Commun. 4:1595 doi: 10.1038/ncomms2596 (2013).